A plasma-treated chalcogenide switch device for stackable scalable 3D nanoscale memory Stackable select devices such as the oxide p-n junction diode and the Schottky diode (one-way switch) have been proposed for non-volatile unipolar resistive switching devices; however, bidirectional select devices (or two-way switch) need to be developed for bipolar resistive switching devices. Here we report on a fully stackable switching device that solves several problems including current density, temperature stability, cycling endurance and cycle distribution. We demonstrate that the threshold switching device based on As-Ge-Te-Si material significantly improves cycling endurance performance by reactive nitrogen deposition and nitrogen plasma hardening. Formation of the thin Si 3 N 4 glass layer by the plasma treatment retards tellurium diffusion during cycling. Scalability of threshold switching devices is measured down to 30 nm scale with extremely fast switching speed of ~2 ns. The two basic components of random access memory devices are the select switch and storage node. It is required to improve the performance of both of these elements to achieve terabit density memory. Furthermore, both components will be required to be compatible with technologies such as three-dimensional (3D) cell stacking, multi-level cell, endurance and scaling for future memory and switch devices [1] , [2] . Resistive random access memory has been considered to be one of the most promising candidates to overcome scaling limits of the conventional memory due to its scalability, data retention (non-volatility), fast switching speed and low power consumption [3] , [4] , [5] , [6] , [7] , [8] , [9] , [10] , [11] , [12] , [13] , [14] , [15] . In a high-density memory system such as dynamic random access memory, a select device is required to suppress sneak current paths [3] , [8] , [9] . Current select devices have been Si-based transistors to obtain sufficient on-current density and reliability. However, the three-terminal Si transistors are not suitable for 3D crossbar stacked structure due to their high processing temperature and difficulty in both scaling and stacking [8] , [9] . Recently, various bidirectional select devices, for instance the varistor-type switch [16] and mixed-ionic-electronic-conduction device [17] have been proposed for bipolar resistive memory applications. The threshold switching (TS) devices are able to overcome the previous limitations by imitating bidirectional diode-like behaviour while being composed of a single compound and providing sufficient current density. Initially, oxide materials such as V 2 O 5 (refs 18 , 19 ) and NiO 2 (ref. 20 ) as well as several chalcogenide materials [21] , [22] have been investigated as TS materials. The chalcogenide material, As-Te-Ge-Si, despite its good TS characteristics, has had key issues on degradation with repeated cycling and reliability at postprocessing temperatures of 500–600°C [21] , [23] . In this report, we present two nitrogen (N 2 ) processes, reactive N 2 sputtering and plasma hardening, which together form a thin, highly crosslinked glass Si 3 N 4 -based barrier that suppresses Te diffusion in the chalcogenide film, leading to dramatic improvement on its endurance and switching distribution. We believe that a similar treatment is applicable to any materials in which elemental diffusion limits reliability and cycle-to-cycle distribution. Especially, the introduction of reactive N 2 during deposition improves the thermal stability of the chalcogenide glass, allowing for the memory node and switch device to be integrated into a single stack in contrast with previous studies that utilized a wire-bonded connection or another external method of combining switching devices and memory nodes [8] , [19] , [24] . Resistive memory and TS devices Due to the single material composition and ease of deposition onto arbitrary substrates, TS devices are ideal for stacked 3D memory structures, as shown in Fig. 1a . The scheme presented here stacks a memory element with a switch element between crossbar metal electrodes, which allows the highest cell geometric density. We demonstrate the I-V characteristics of the As-Te-Ge-Si-N switch and the TaO y /Ta 2 O 5–x memory node for (0.5 um) 2 cell sizes, respectively, in Fig. 1b,c . 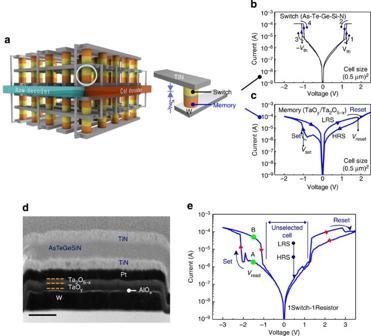Figure 1:TaOy/Ta2O5–xresistive switching and As-Te-Ge-Si-N TS devices. (a) Idealized schematic of 3D-stacked memory structure using switch and memory element in crossbar array structure with enlarged view of memory cell. (b)I-VTS operation of the switch device (As-Te-Ge-Si-N) in the crossbar array. (c)I-Vnon-volatile switching operation of the memory device (TaOy/Ta2O5–x) in the crossbar array. (d) A cross-sectional TEM image of the 1S–1R with W/AlOx/TaOy/Ta2O5–x/Pt/TiN/As-Te-Ge-Si-N/TiN-stacked structure. Scale bar, 100 nm. (e)I-Vcharacteristics of combined switch and memory device structure described with reduced leakage current at below ±1 V (readout margin for data reading in crossbar array). In the switch device, we observe a volatile TS with threshold voltage of ±1 V. Meanwhile, the memory device shows non-volatile bipolar resistive switching between a high resistance state (HRS) and a low-resistance state (LRS) with the V set =−1 V and V reset =+2 V. Figure 1: TaO y /Ta 2 O 5–x resistive switching and As-Te-Ge-Si-N TS devices. ( a ) Idealized schematic of 3D-stacked memory structure using switch and memory element in crossbar array structure with enlarged view of memory cell. ( b ) I-V TS operation of the switch device (As-Te-Ge-Si-N) in the crossbar array. ( c ) I-V non-volatile switching operation of the memory device (TaO y /Ta 2 O 5–x ) in the crossbar array. ( d ) A cross-sectional TEM image of the 1S–1R with W/AlO x /TaO y /Ta 2 O 5–x /Pt/TiN/As-Te-Ge-Si-N/TiN-stacked structure. Scale bar, 100 nm. ( e ) I-V characteristics of combined switch and memory device structure described with reduced leakage current at below ±1 V (readout margin for data reading in crossbar array). Full size image Figure 1d shows a cross-sectional transmission electron microscopy image of the stacked structure that combines our memory and select device. The TaO y /Ta 2 O 5–x bilayer memory element has been previously demonstrated to show non-volatile high endurance up to 10 12 and considered to be an appropriate material for the study of switch elements [3] . The structure begins with the bottom W electrode onto which a thin 2 nm buffer layer is deposited by atomic layer deposition. This AlO x buffer layer is used to reduce excessive voltage drop across the switch and memory node when they are both in their respective LRS [3] . In addition, the thin AlO x layer suppresses any chemical reaction between the W electrode and the memory node layer [3] . Next, the TaO y (20 nm)/Ta 2 O 5–x (10 nm) bilayer memory stack is deposited as a storage element. The middle electrode is a Pt/TiN double layer contacted to the appropriate sides for optimal switching [3] . The As-Te-Ge-Si-N chalcogenide TS layer is then deposited. To form a highly crosslinked glass Si 3 N 4 -based barrier using the Si within the switching material, we subsequently use a N 2 plasma-hardening process on the deposited chalcogenide layer. Finally, the TiN top electrode is formed to complete the stacked device. Figure 1e shows the I-V characteristics of the combined one switch-one resistor (1S–1R) stack structure ( Supplementary Fig. S1 also shows the multiple cycling to demonstrate the combined switching concept). For combined operation of the switch and resistor, the set and reset voltages V set and V reset of the resistor should ideally both be larger than the threshold voltage of the switch device ± V threshold . The reading operation is performed at V read of −1.5 V where the largest on/off ratio occurs. When the resistance device is in the off-state, the current value at A will be read, whereas when the resistance is in the on-state, the current value B will be read. In both previous cases, the reading voltage is chosen so the specific switch device is turned on, whereas adjacent switch devices in a theoretical array are kept off. In both reading cases, the switch is turned on so that the non-volatile memory device determines the reading current. As the memory is scaled down and better materials and processes are developed to reduce the on-state (and off-state current), the reading current will correspondingly decrease. As-Ge-Te-Si and As-Ge-Te-Si-N switch devices To write to the 1S–1R device V set of −2 V is applied, which turns on both the switch device and sets the resistance device to the LRS. Meanwhile, for the erase operation of the 1S–1R device, a V reset of +3 V is applied, which turns on the switch device and sets the resistance device to the HRS. To integrate further devices in a stack, we could start W deposition again and duplicate the structure repetitiously. One should note that the highest temperature during stack fabrication occurs for the TaO y /Ta 2 O 5–x memory storage layer at ~400°C. For pristine As-Ge-Te-Si switches, without reactive N 2 , severe thermal degradation takes place as compared in Fig. 2a,b . After annealing As-Ge-Te-Si switches at 500°C in vacuum the device failed after just a few cycles. In addition, the optimal N 2 amount was sensitive down to just 1 sccm during N 2 reactive sputtering. 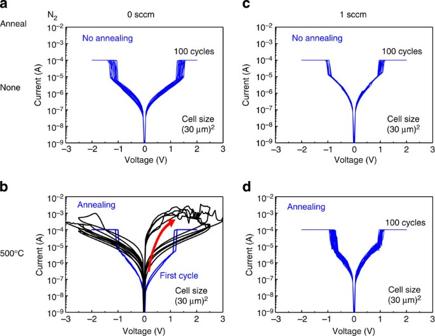Figure 2: Comparison of electrical cycling between both annealed and unannealed As-Ge-Te-Si and As-Ge-Te-Si-N switch devices. (a) As-deposited As-Ge-Te-Si, (b) annealed As-Ge-Te-Si, (c) as-deposited As-Ge-Te-Si-N and (d) annealed As-Ge-Te-Si-N switch devices. These data show 100 switching cycles for each device exceptb. Figure 2c,d confirms that with 1 sccm for reactive N 2 introduced, although the initial properties were relatively unaffected, the thermal stability was greatly improved and cycling with a good distribution was demonstrated. Further increasing the N 2 amount to 2 sccm slightly degraded the switching distribution, whereas past 10 sccm the As-Ge-Te-Si-N film did not show reliable switching ( Supplementary Fig. S2 ). The reactive N 2 process allowed for a fully integrated 1S–1R device to be investigated and properties of the stackable cell to be verified. Further elucidation is required into the role of N 2 in the films, which acts to thermally stabilize the chalcogenide glass; however, it may be related to Si 3 N 4 within the film, which retards crystallization of the chalcogenide material and affects the diffusivity of Te [23] ; ( Supplementary Fig. S3 ). Figure 2: Comparison of electrical cycling between both annealed and unannealed As-Ge-Te-Si and As-Ge-Te-Si-N switch devices. ( a ) As-deposited As-Ge-Te-Si, ( b ) annealed As-Ge-Te-Si, ( c ) as-deposited As-Ge-Te-Si-N and ( d ) annealed As-Ge-Te-Si-N switch devices. These data show 100 switching cycles for each device except b . Full size image The I-V measurements of the complete 1S–1R structure in stacked cell, namely, W/AlO x /TaO y /Ta 2 O 5–x /Pt/TiN/As-Te-Ge-Si-N/TiN are shown in Fig. 1e to confirm that processing did not cause damage to the device. The change from HRS to LRS (set) occurs at −2.2 V, whereas the opposite process (reset) occurs at +2.8 V. At below ±1 V, the TS device is off so that no programming can occur. The behaviour of the switch and the memory layers are clearly demonstrated in a single integrated stack. It is important to note that the leakage current level at a voltage of below ±1 V (off state of TS device) determines the possible array size for memory that can be achieved as stray current paths must be blocked (this is further explained by using a 1/3-V programming method in the Supplementary Fig. S4 ). More information regarding memory array size and the stray leakage path issues are presented in the Supplementary Fig. S5 . The on/off ratio of the combined memory cell was about two orders of magnitude as read in the negative biasing conditions at −1.5 V, as shown in Fig. 1e (green circles). XPS analysis and scalability of As-Ge-Te-Si-N switch devices We further investigated the properties of the select device and the effects of the previously mentioned N 2 plasma-hardening process, which led to a significant improvement in cycle-to-cycle switching distribution. The depth profiles of X-ray photoelectron spectroscopy (XPS) were used to analyse the film composition. The depth profile of a pristine As-Te-Ge-Si-N layer (with reactive N 2 ) is shown in Fig. 3a . Annealed at 500°C, this sample was then electrically switched 1,000 times as shown in Fig. 3b . The degradation with continuous switching was apparent as the off-state resistance was reduced by almost two orders of magnitude. The switching voltage also decreased on average while additionally having a wide distribution even between consecutive cycles. After cycling, we performed another XPS depth profile and were able to observe a significant change to the composition. Especially striking was the immense diffusion of the Te layer as shown in Fig. 3c from XPS results. Previous models of TS in As-Te-Ge-Si-N have proposed that Te acts as the key material for switching because the trap sites in the deep level were converted to the shallow level in the presence of high fields [21] , [25] , [26] , [27] , [28] , [29] . The exact effects of Te diffusion have not been considered at this time; however, it probably seems to be related to both the wide distribution and degraded device resistance properties. Before deposition of the top TiN electrode, another sample ( Fig. 3d ) was prepared with our N 2 plasma-hardening treatment. Highly energized N 2 atoms have been previously shown to increase the degree of crosslinking in Si 3 N 4 glasses [30] , which would retard diffusion across the region due to reduction of defect sites [23] . After annealing at 500°C, we run the N 2 plasma-treated device for 1,000 cycles as shown in Fig. 3d . The improvement in switching distribution was clear and there was almost no discernible degradation of the off-state resistance. The depth profile in XPS of the N 2 plasma-treated sample in Fig. 3e displays a clear difference between the untreated and the treated samples after cycling. In the N 2 -treated sample, the Te region is only slightly reduced in comparison to the pristine sample of Fig. 3a . The depth profile in XPS also showed the higher N 2 concentrations near the interface between the electrode and switching layer (~30 min of sputtering time as shown in Fig. 3e ) for the plasma-treated sample. However, it should be noted that an exact analysis of N 2 content is difficult due to the existence of the TiN top electrode. We used the trap-limited conduction model [21] to relate the off-state current with the total trap density and the average trap distance ( Supplementary Fig. S6 ) within the As-Te-Ge-Si-N-deposited films and indeed the model indicated that trap density decreased from 1.5 × 10 18 down to 4 × 10 17 cm −3 after plasma treatment and annealing, as shown in Supplementary Fig. S6 . 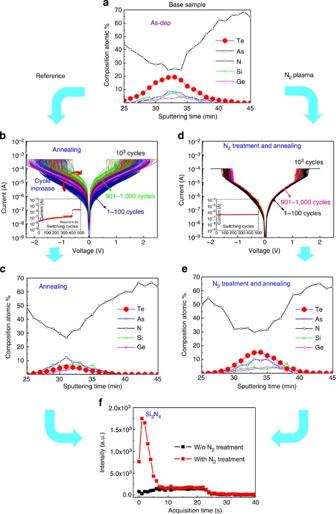Figure 3:XPS depth profiling. (a) Profiled as-deposited As-Ge-Te-Si-N device (with reactive N2). (b) Electrical cycling for 1,000 cycles ((0.5 um)2cell size) and (c) XPS depth profile of the annealed and cycling of as-deposited As-Ge-Te-Si-N device. (d) Electrical cycling for 1,000 cycles ((0.5 um)2cell size) and (e) XPS depth profile of the annealed N2plasma-treated As-Ge-Te-Si-N device. (f) SIMS profile showing formation of Si3N4in the N2plasma-treated device. Insets inbanddshow the change in off-state current by switching cycle. Figure 3: XPS depth profiling . ( a ) Profiled as-deposited As-Ge-Te-Si-N device (with reactive N 2 ). ( b ) Electrical cycling for 1,000 cycles ((0.5 um) 2 cell size) and ( c ) XPS depth profile of the annealed and cycling of as-deposited As-Ge-Te-Si-N device. ( d ) Electrical cycling for 1,000 cycles ((0.5 um) 2 cell size) and ( e ) XPS depth profile of the annealed N 2 plasma-treated As-Ge-Te-Si-N device. ( f ) SIMS profile showing formation of Si 3 N 4 in the N 2 plasma-treated device. Insets in b and d show the change in off-state current by switching cycle. Full size image Further investigation with secondary ion mass spectroscopy as shown in Fig. 3f reveals that N 2 plasma treatment creates a thin Si 3 N 4 layer on the surface of As-Te-Ge-Si -N switch material. In addition, high-temperature XRD measurements for N 2 plasma treatment show that the amorphous phase are well maintained at over 600°C ( Supplementary Fig. S7 ). The contrast between the as-deposited and plasma-treated samples from the secondary ion mass spectroscopy data concludes as follows; the formation of a Si 3 N 4 barrier layer at the surface and SiN bonding by plasma treatment retard Te diffusion, which in turn leads to improved cycle-to-cycle disturbance. Aforementioned current density across the switch device must be sufficient for switching the TaO y /Ta 2 O 5–x memory cell into the HRS and the LRS. We found low-resistance state current to be sufficient by drastically shrinking switch devices from (100 μm) 2 all the way down to (30 nm) 2 cell size to determine the scaling behaviour of the As-Ge-Te-Si-N switch devices. A 500-nm device array fabricated by photolithography is shown in Fig. 4a and a single (30 nm) 2 cell-size device fabricated by electron beam lithography is shown in Fig. 4b . 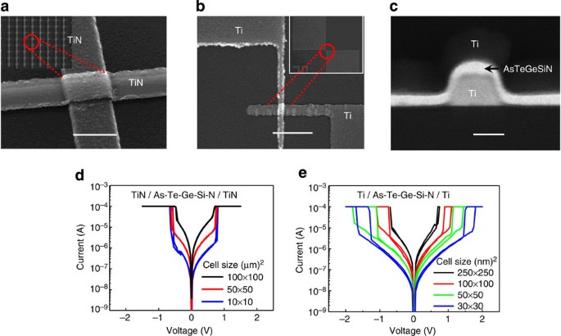Figure 4:Device scalability demonstrated inscanning electron microscopyandscanning transmission electron microscopyimages. (a) Scanning electron microscopy (SEM) image of (500 nm)2cell size with the inset showing an 8 × 8 array of 500 nm switch devices. Scale bar, 500 nm. (b) SEM image of a single (30 nm)2cell-size device. The inset shows a shrunk image with top and bottom electrodes. Scale bar, 100 nm. (c) Cross-sectional scanning transmission electron microscopy of (30 nm)2cell size. Scale bar, 30 nm. (d) Switching behaviour of (100 um)2, (50 um)2and (10 um)2cell-size devices with TiN electrodes. (e) Switching behaviour of (250 nm)2, (100 nm)2, (50 nm)2and (30 nm)2cell-size devices with Ti electrodes. Figure 4c shows cross-sectional scanning transmission electron microscopy of (30 nm) 2 cell size with Ti electrodes and As-Te-Ge-Si-N switch material. Measurements in Fig. 4d were done on cell-size devices of (100 μm) 2 , (50 μm) 2 and (10 μm) 2 , as described in Fig. 4a . Meanwhile, cell-size devices of (250 nm) 2 , (100 nm) 2 , (50 nm) 2 and (30 nm) 2 in Fig. 4e were measured in a device structure as shown in Fig. 4b . Ti electrodes were much less optimized for our devices than the TiN electrodes we were able to use for devices fabricated using photolithography. In fact, the leakage current for test devices fabricated at 500 × 500 nm 2 cell size showed that Ti electrodes increased the leakage current by almost two orders of magnitude for switches in the off-state ( Supplementary Fig. S8 ). Figure 4: Device scalability demonstrated in scanning electron microscopy and scanning transmission electron microscopy images. ( a ) Scanning electron microscopy (SEM) image of (500 nm) 2 cell size with the inset showing an 8 × 8 array of 500 nm switch devices. Scale bar, 500 nm. ( b ) SEM image of a single (30 nm) 2 cell-size device. The inset shows a shrunk image with top and bottom electrodes. Scale bar, 100 nm. ( c ) Cross-sectional scanning transmission electron microscopy of (30 nm) 2 cell size. Scale bar, 30 nm. ( d ) Switching behaviour of (100 um) 2 , (50 um) 2 and (10 um) 2 cell-size devices with TiN electrodes. ( e ) Switching behaviour of (250 nm) 2 , (100 nm) 2 , (50 nm) 2 and (30 nm) 2 cell-size devices with Ti electrodes. Full size image The I-V behaviour across seven orders of devices size did not change significantly and the TS was observed across all devices. Interestingly, the on-current did not scale with device size up to the given 100 μA compliances due to the filamentary nature of on-state conduction, indicating that sufficient current can be provided for electrical switching by TS switch devices. Supplementary Fig. S9 shows that even for small sizes the on-current remains the same as for larger ones. For the 30 × 30 nm 2 cell, the current density of 1.1 × 10 7 A cm −2 was achieved, which approaches on-current density values of single-crystalline Si vertical diode at 90 nm technology node [31] . The mechanism behind filamentary TS is related to local current path formation at the threshold voltage by the electro-thermal model, which has been previously described by Kostylev [32] , [33] . Due to the highly conductive filamentary paths nature of the TS device, which is expected to be of the order of 3 nm diameter [32] , [33] , even devices down to 30 nm can provide 100 uA current in the LRS. Meanwhile, we measured the switching speeds for 30 nm-sized cells with external load resistances of 10 and 50 Ω for impedance matching. The input pulse and response pulse are shown in Fig. 5a . The input pulse used was 3.4 V with a pulse width of 100 ms and a rising/falling time of 1 ms. Our best results for device switching speeds showed extremely fast switching speeds for both transitions into on- and off-states at 4 ns and under 2 ns, as shown in Fig. 5b,c , respectively. It should be noted that improved manufacturing methods will be required before a large-scale array could attain 4 ns switching speeds. The measured switching speeds were similar to those proposed by the electro-thermal model [33] probably indicating that plasma treatment of our samples did not affect the primary switching mechanism. Further direct current (DC) measurements showing on/off ratio 1.5 orders of magnitude and several cycles of switching for (30 nm) 2 and (70 nm) 2 cell sizes are presented in the Supplementary Fig. S10 . 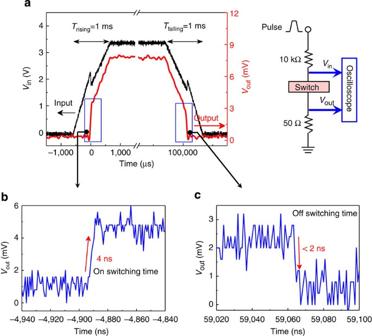Figure 5: Measured switching speed of As-Te-Ge-Si-N 30 nm-sized switch device. (a) Real-time oscilloscope response measuring switching speed with external circuit schematics used detailed on right. (b) Zoomed-in response at the instant from off-state to on-state. Switching time was 4 ns. (c) Zoomed-in response at the instant from on-state to off-state. Switching time was under 2 ns. Figure 5: Measured switching speed of As-Te-Ge-Si-N 30 nm-sized switch device. ( a ) Real-time oscilloscope response measuring switching speed with external circuit schematics used detailed on right. ( b ) Zoomed-in response at the instant from off-state to on-state. Switching time was 4 ns. ( c ) Zoomed-in response at the instant from on-state to off-state. Switching time was under 2 ns. Full size image Endurance of our switch devices for (30 um) 2 and (500 nm) 2 cells did not show any degradation up to 10 8 switching cycles as shown in Fig. 6 . For 30 um cells, we used on-current values limited by compliance current, whereas 500 nm cells were limited using an external 4 kΩ load resistance, as shown in Fig. 6a . The effect of load resistance for measurement of on-current is described in Supplementary Fig. S11 . 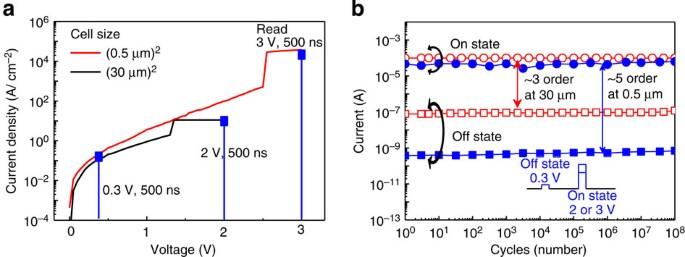Figure 6: Cycling endurance in As-Ge-Te-Si-N switch devices. (a) DCI-Vmeasurement of the (30 um)2cell-size device using compliance current and (500 nm)2cell-size device using external 4 kΩ load resistance. Pulse is measured with reading voltages for on/off-states indicated by drop lines. (b) Cycling endurance up to 108shown for (30 um)2and (500 nm)2cell-size devices. The inset shows a diagram of voltage pulses for testing this scheme. Figure 6a demonstrates that the DC measurement behaviour of both cells and the pulse measurement parameters (voltages and widths) are shown at the appropriate points. A 0.3-V, 500-ns pulse was used to read off-state in both cell sizes, whereas a 2-V, 500-ns pulse was used to measure on-state in the (30 um) 2 cell, and a 3-V, 500-ns pulse was used to measure the on-state in the (500 nm) 2 cell, respectively. We cycled our devices for up to 10 8 cycles as observed in Fig. 6b . The on/off ratio was ~3 orders and ~5 orders for (30 um) 2 and (500 nm) 2 cells, respectively. As expected, the increased on-current density for smaller cell sizes leads to higher on/off ratios for the smaller cell sizes. Finally, we confirmed switching behaviour of cycling endurance down to 50 ns ( Supplementary Fig. S12 ), which is appropriate for oxide memory materials for high-speed operation [3] . Figure 6: Cycling endurance in As-Ge-Te-Si-N switch devices. ( a ) DC I-V measurement of the (30 um) 2 cell-size device using compliance current and (500 nm) 2 cell-size device using external 4 kΩ load resistance. Pulse is measured with reading voltages for on/off-states indicated by drop lines. ( b ) Cycling endurance up to 10 8 shown for (30 um) 2 and (500 nm) 2 cell-size devices. The inset shows a diagram of voltage pulses for testing this scheme. Full size image In summary, we demonstrated a switching device based on As-Ge-Te-Si material, which is significantly improved by two N 2 processes: reactive N 2 during deposition and N 2 plasma hardening. The introduction of N 2 in the above two-step processing enables a stackable and thermally stable device structure, allowing integration of switch and memory devices. Furthermore, the thin Si 3 N 4 glass layer formed by the plasma process retards Te diffusion during cycling leading to highly improved electrical performance. The thermal budget of N 2 plasma-treated As-Ge-Te-Si-N in postprocessing is sufficient for stacked structures, overcoming a previous limitation of chalcogenide switching materials. In addition, electrical performance was measured down to 30 nm scale with extremely fast switching speed of ~2 ns and proved to be satisfactory for nanoscale memory applications in high-density integration. Electrical pulse measurements The DC electrical measurements of test cells were performed by using an Agilent 4156C Semiconductor Parameter Analyzer. Pulse measurements for cycling endurance were conducted by an Agilent 81110 A pulse generator and Tektronix oscilloscope (6 GHz). For cycling endurance measurements, an external load resistance was serially connected between the device and the analyser. Uniformity of samples across a 150-mm wafer was measured using DC measurements to cycle respective devices 100 times each ( Supplementary Fig. 13 ). Preparation of memory and switch devices We fabricated both W/AlO x /TaO y /Ta 2 O 5–x /Pt resistor structures as memory devices and TiN/As-Te-Ge-Si-N/TiN or Ti structure as bidirectional switch devices. All films were deposited by using reactive DC magnetron sputtering based on the respective metal target. For the fabrication of memory devices, W bottom electrode was deposited. Next, the TaO y layer is deposited and the insulating Ta 2 O 5–x layer was subsequently formed by placing our samples in an O 2 plasma oxidation chamber used for atomic layer deposition and capped by top Pt electrode. After that, the TiN (Ti for cell sizes below 250 nm) switch contact was formed by reactive sputter of a Ti target in a mixture of N 2 and Ar. Then, a 40-nm switch layer of As-Ge-Te-Si-N was deposited using reactive sputter of an As-Te-Ge-Si target again in a mixture of N 2 and Ar gas, and a N 2 plasma treatment was formed and capped with the top TiN or Ti electrode (for cell sizes below 250 nm). E-beam lithography was used to define crossbar cell structures of switch devices from 250 to 30 nm sizes. First, a two-layered electroresist fabrication process was used to create Ti bottom electrode lines (40 nm thick) on the 500-nm thick SiO2 substrates. The two electroresist layers were composed of ZEP-520A7 from ZEONREX Electronic Chemicals on top of Lift-off-Resist 1A (LOR1A) from Microchem Corp. This method was used to define a more precise cell structure to achieve accurate measurements and higher device yields. Top Ti deposition was performed using E-beam evaporation after pattering the bottom lines by E-beam lithography and then using a lift-off method. Device sizes from (0.5 um) 2 and above were fabricated similar to E-beam samples; however, conventional projection photolithography was used. Annealing conditions for the experiments presented in Fig. 2 were performed within the sputtering chamber. First the chamber was pumped down to a base pressure of 10 −7 Torr and the substrate holder temperature was increased to 500°C. The samples were annealed from 15 to 30 min and then removed. In addition, annealing in N 2 ambient at 30 mTorr under the same temperature was performed, however, device performance for both reactive N 2 devices and pristine devices did not show any difference from those of vacuum-annealed samples. Trap-limited conduction model We performed the modelling for off-state conduction based on the trap-limited conduction (TLC) mechanism [21] for an As-Te-Ge-Si-N chalcogenide glass. From the TLC mode1 (ref. 21 ), the current ( I ) can be described as where q is the elementary charge, A is the area of the contact, N T is the integral of the trap distribution in the gap above the Fermi level, Δ z is the average distance between two traps, τ 0 is the characteristic attempt-to-escape time for the trapped electron (~10 −13 s), E C is the energy at the conduction band edge, E F is the Fermi level, V A is the applied voltage and u a is the amorphous chalcogenide thickness (~50 nm). As the real trap distribution in the chalcogenide material is generally not known, we will neglect the inaccuracies of equation 1 for E C and E F and will treat N T as an effective trap concentration. By using the TLC model [21] , we extracted the total trap density ( N T ) and inter-trap distance (Δ z ) at experimental switching data (10 3 cycles) of various process conditions as shown in Supplementary Fig. S6 . Compared with the as-deposited sample, the change in trap density and distance of N 2 -treated and annealed one was suppressed, which means trap density and distance are strongly related with Te loss. How to cite this article: Lee, M.-J. et al. A plasma-treated chalcogenide switch device for stackable scalable 3D nanoscale memory. Nat. Commun. 4:2629 doi: 10.1038/ncomms3629 (2013).